A reversible long-life lithium–air battery in ambient air Electrolyte degradation, Li dendrite formation and parasitic reactions with H 2 O and CO 2 are all directly correlated to reversibility and cycleability of Li–air batteries when operated in ambient air. Here we replace easily decomposable liquid electrolytes with a solid Li-ion conductor, which acts as both a catholyte and a Li protector. Meanwhile, the conventional solid air cathodes are replaced with a gel cathode, which contacts directly with the solid catholyte to form a closed and sustainable gel/solid interface. The proposed Li–air cell has sustained repeated cycling in ambient air for 100 cycles (~78 days), with discharge capacity of 2,000 mAh g −1 . The recharging is based largely on the reversible reactions of Li 2 CO 3 product, originating from the initial discharge product of Li 2 O 2 instead of electrolyte degradation. Our results demonstrate that a reversible long-life Li–air battery is attainable by coordinated approaches towards the focal issues of electrolytes and Li metal. Lithium-air batteries integrate the most electronegative and lightest metal of Li with the inexhaustibly ambient O 2 , hence attracted intensive attentions due to the main application driving interest in transportation [1] . However, the inherent Li–O 2 couple is also double-edged to two critical challenges in cell operation. (1) Superoxide anion radical species (O 2 − ) is formed during O 2 reduction, which reacts with majority of aprotic liquid electrolytes such as alkyl carbonate, acetonitrile and dimethylformamide [2] , [3] , [4] , [5] . (2) Li dendrite formation during repeated cycling leads to severe safety issue [6] , impressed by the explosion hazards [7] , and Li metal reacts strongly with the moisture and CO 2 if operating in air. So far, intensive efforts on electrolyte screening have identified the tetra(ethylene)glycol dimethyl ether [8] , [9] and the dimethyl sulfoxide [10] , [11] as relative stable electrolytes against O 2 − , and achieved substantial improvements on cell reversibility in pure O 2 . However, these liquid electrolytes are still subject to some restrictions, for instance, dimethyl sulfoxide has high volatility and is unstable with Li metal [11] ; the stability of ether-based electrolytes were still ambiguous according to several reports [12] , [13] , [14] . Most importantly, there is still no evidence that the improved Li–O 2 cells are able to operate in ambient air for long period. As an alternative approach, we replaced liquid electrolytes with a solid conductor of Li 1.35 T 1.75 Al 0.25 P 2.7 Si 0.3 O 12 (LTAP) to circumvent the decomposition problem of liquid electrolytes primarily. The LTAP has been commonly utilized as a separator for hybrid electrolytes [15] , [16] , [17] , [18] . However, herein it can act as catholyte directly, assisted by a neoteric gel air cathode: crosslinked network gel (CNG) consisting of single-walled carbon nanotubes (SWNTs) and ionic liquid (IL) of 1-ethyl-3-methylimidazolium ([C 2 C 1 im]) bis(trifluoromethylsulfonyl)imide ([NTf 2 ]) ( [19] . The structure of the proposed Li–air cell in this study is illustrated in Fig. 1 . The CNG possesses superior ‘three-dimensional tri-continuous passages of electron, ion and oxygen’, which enables the three-phase cathodic reaction occurring independent of liquid electrolyte permeation. Additionally, its gel characterization is desirable to establish a closed and sustainable interface with solid catholyte, in contrast to solid cathodes [20] . Furthermore, taking the protection of LTAP for Li metal into account, the short-circuit touch of Li dendrite with air cathode, and the parasitic reactions between Li metal and air can be avoided. 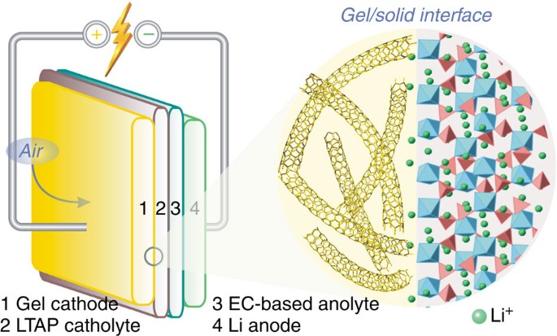Figure 1: Schematic illustration of the proposed Li–air cell. Detailed configuration is described in the Methods section. Figure 1: Schematic illustration of the proposed Li–air cell. Detailed configuration is described in the Methods section. Full size image In this study, we show that the proposed Li–air cell is capable of cycling in ambient atmosphere for a long period. On discharging, the initial discharge product is hexagonal polycrystalline Li 2 O 2 , which changes into LiOH, and then Li 2 CO 3 due to chemical reactions with moisture and CO 2 in ambient air. During charging, the predominant discharge product of Li 2 CO 3 decomposes electrochemically in the gel air cathode to achieve a reversible cycling process. Our results provide a proof of Li–air batteries operated in ambient air. Discharge/charge behaviour with CNG The proposed Li–air cell was attempted firstly under an atmosphere containing pure O 2 with trace of air to assess the influence of tiny moisture and CO 2 , and afterwards, operated under real ambient air. 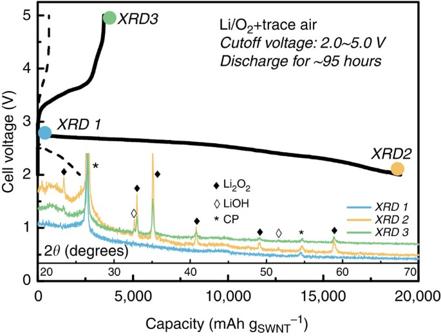Figure 2: Discharge/charge performance and XRD analysis of Li–air batteries in O2with a trace of air. Discharge/charge curves of the cells with SWNTs/IL CNG (continuous line) and mixture (broken line) at 200 mA gSWNT−1in 1 atm pure O2with a trace of air. The inset shows the corresponding XRD patterns of the CNG air electrode in its pristine state (XRD 1), after discharged to 2 V (XRD 2) and then recharged to 5 V (XRD 3). Carbon paper (CP) was used as the current collector of cathode. Figure 2 shows the discharge/charge behaviour of the proposed Li–air cell in pure O 2 with a trace of air at first. In terms of the capacity based on SWNTs, the cell with SWNTs/IL CNG exhibit 19,050 mAh g −1 , over eight times of 2,210 mAh g −1 for the cell with SWNTs and IL mixture (before gelation). The SWNTs, as the electron passage, provide the total number of surface sites for discharge products deposition. Therefore, the discharge results represent the superior accommodating capability of the untangled SWNTs for discharge products. By virtue of the significant quantity of discharge products, all of the strong peaks within 20°~60°, agreement with Li 2 O 2 X-ray powder diffraction (XRD) file (PDF no. 73–1640), have been identified at the discharge terminal (XRD 2). The diffraction is indexed to hexagonal crystal structure Li 2 O 2 , which is well consistent with the TEM analysis of discharged oxygen electrode [21] . Additionally, weak LiOH peaks are also observed, due to tiny moisture in trace of air. Further X-ray photoelectron spectroscopy (XPS) probe for surface species confirms the presence of slight Li 2 CO 3 ( Supplementary Fig. S1 ), which may come from the reaction of Li 2 O 2 with trace of air, or the reaction at the SWNTs-Li 2 O 2 interface to form a monolayer of Li 2 CO 3 ( [22] , [23] ). However, an unexpected phenomenon happened that the Li–air cell was unable to be totally recharged, exhibiting merely 18% of the discharge capacity. In consistent with this observation, the Li 2 O 2 peaks (see inset of Fig. 2 ) were still in presence at the recharge terminal (XRD 3), but the LiOH peaks have almost disappeared. In impedance spectra, a new semicircle occurred after discharged ( Supplementary Fig. S2 ). This semicircle may reflect a change of charge transfer resistance related to the insulation of Li 2 O 2 products [24] . Figure 2: Discharge/charge performance and XRD analysis of Li–air batteries in O 2 with a trace of air. Discharge/charge curves of the cells with SWNTs/IL CNG (continuous line) and mixture (broken line) at 200 mA g SWNT −1 in 1 atm pure O 2 with a trace of air. The inset shows the corresponding XRD patterns of the CNG air electrode in its pristine state (XRD 1), after discharged to 2 V (XRD 2) and then recharged to 5 V (XRD 3). Carbon paper (CP) was used as the current collector of cathode. Full size image Analysis of discharge/charge process To clarify the reason of partially recharged, the discharge capacity was limited to 1,000 mAh g −1 , and then recharged ( Fig. 3a ). The Li–air cell shows a complete unavailability in recharge until the 14th cycle, in which and in particular the subsequent 15th and 16th cycles, the partial recharge gradually appears. The recharge curves exhibit the similar overpotential with that in Fig. 2 . It suggests that the LiOH was generated upon Li 2 O 2 at the terminal stage of discharge, which subsequently recharged but Li 2 O 2 remained. This phenomenon can be understood by elucidating the discharge–charge process thoroughly. 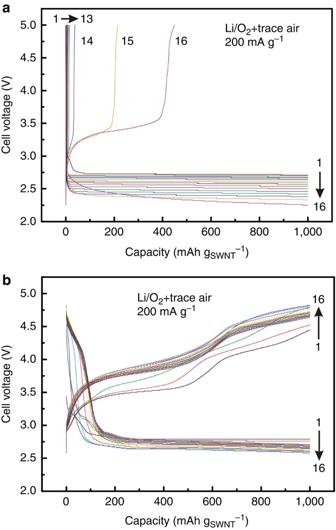Figure 3: Comparison of discharge/charge curves of Li–air batteries with CNG and Li salt-modified CNG. (a) Discharge/charge curves of the cell with CNG under a capacity limitation of 1,000 mAh gSWNT−1. (b) Discharge/charge curves of the cell with Li salt-modified CNG. The tests were carried out in pure O2with a trace of air. Figure 3: Comparison of discharge/charge curves of Li–air batteries with CNG and Li salt-modified CNG. ( a ) Discharge/charge curves of the cell with CNG under a capacity limitation of 1,000 mAh g SWNT −1 . ( b ) Discharge/charge curves of the cell with Li salt-modified CNG. The tests were carried out in pure O 2 with a trace of air. Full size image The following equations show the speculated primary reactions of the Li–air cell with the LTAP catholyte and the CNG gel air cathode in ambient air: Li + +O 2 +e − →LiO 2 oxygen reduction reaction (ORR) (1) 2LiO 2 →Li 2 O 2 +O 2 (2) 2Li 2 O 2 +2H 2 O→4LiOH+O 2 (3) 2LiOH+CO 2 →Li 2 CO 3 +O 2 (4) Li 2 O 2 →2Li + +O 2 +2e − oxygen evolution reaction (OER) (5) 4LiOH→4Li + +O 2 +2H 2 O+4e − OER (6) 2Li 2 CO 3 →4Li + +O 2 +2CO 2 +4e − OER (7) As reported previously [3] , [10] , the discharge of the Li–air cell is initiated with the transient formation of O 2 − , which is a highly reversible one-electron process involving the O 2 /O 2 − couple (O 2 +e − ↔O 2 − ). The O 2 − is a very powerful nucleophile, and tends to attack positively charged components of any organic species present [25] , nevertheless, owing to the soft acidity of the [C 2 C 1 im] + imidazolium cation, strong O 2 − ···[C 2 C 1 im] + ion-pairs are preferred via the nucleophilic addition of O 2 − to [C 2 C 1 im] + ( [26] , [27] ), thereby stabilized the O 2 − in the CNG (O 2 +[C 2 C 1 im] + ↔O 2 − ···[C 2 C 1 im] + ). Next, if Li + cation, a hard Lewis acid, is introduced, it is able to promote disproportionation of O 2 − to peroxide and O 2 ( [28] ). In the case of Fig. 3a , once the Li + ions transported from the LTAP into the CNG along its ions passage, they incorporated with all of the superoxides, including that in O 2 − ···[C 2 C 1 im] + ion-pair and the newly electrogenerated ones, to form LiO 2 , and then decomposed via disproportionation to produce the Li 2 O 2 (reactions (1) and (2)). This reaction process obeyed the Hard Soft Acid Base theory of Pearson [29] , [30] . The Li 2 O 2 product can be maintained singly for a period because the CNG gel is stable against macro water due to the hydrophobic anchored IL inside [19] . However, some H 2 O molecules in air will still permeate through the oxygen channels to react with Li 2 O 2 and generate LiOH (reaction (3)) ultimately. Compared with Li 2 O 2 , LiOH is facile to dissociate, and thus provides Li + ions, which are indispensable for charging circuit. In another words, the permeated H 2 O has a promoter role (reactions (3) and (6)) for partial Li 2 O 2 decomposition by improving the available Li + ions, which return through the LTAP catholyte, and thus facilitating the charging process. Discharge/charge behaviour with Li salt-modified CNG We attempted to modify the CNG by introducing the Li salt of LiTFSI into the CNG in advance. Figure 3b displays the discharge and charge curves of the Li–air cell with the Li salt-modified CNG. A most exciting observation is the ability to cycle the Li–air cell repeatedly and stably in the presence of Li salt since the first cycle. The cell was cycled for 100 cycles, in which the oxygen reduction reaction and OER potentials of the 50th and 100th cycle was almost same ( Fig. 4 ). The impedance spectra show that the Li salt-modified CNG electrode has a significant reduction in the Warburg resistance related to Li + diffusion ( Supplementary Fig. S3 ). The polarization factors due to the kinetic and diffusion barriers were reported to affect the discharge product distribution greatly [31] . Herein, our results indicated that reducing the diffusion barrier by increasing Li + ions content is an important factor in facilitating the reversible charging process in the gel cathode/solid catholyte interface: (i) The ionic conductivity in the CNG electrode increases with the Li + ions content increasing; (ii) According to Nernst equation, the increasing Li + ions concentration tends to cause the electrode potential of the half-reaction OER (reactions (5)) to be nearer to its equilibrium value. 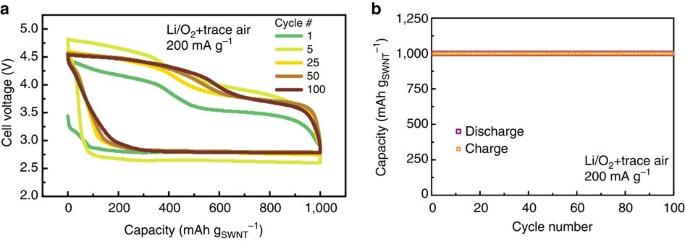Figure 4: Cycling performance of Li–air cell in pure O2with a trace of air. (a) Discharge/charge curves and (b) cycling profiles of the Li–air cell with Li salt-modified CNG under a capacity limitation of 1,000 mAh gSWNT−1for 100 cycles. The tests were carried out in pure O2with a trace of air. Figure 4: Cycling performance of Li–air cell in pure O 2 with a trace of air. ( a ) Discharge/charge curves and ( b ) cycling profiles of the Li–air cell with Li salt-modified CNG under a capacity limitation of 1,000 mAh g SWNT −1 for 100 cycles. The tests were carried out in pure O 2 with a trace of air. Full size image Cycling performance in ambient air The improved Li–air cell with the Li salt-modified CNG was then subjected to operate in ambient air. As seen in Fig. 5 , the discharge capacity reaches 56,800 mAh g −1 , and the recharge capacity is 53,900 mAh g −1 with a high columbic efficiency of 95%, in comparison to the 18% in Fig. 2 . As the current density is 200 mA g −1 , it means that the Li–air cell was operated reversibly for over 550 h to achieve one cycle. According to the corresponding XRD patterns in Fig. 5 , it is unsurprising that majority of the discharge products Li 2 O 2 has changed into Li 2 CO 3 during the long-term discharge (XRD 2) in ambient air. By further comparison with the XRD patterns in Fig. 2 , we can then deduce that the Li 2 O 2 reacted with H 2 O to form LiOH at first, and the LiOH reacted with CO 2 to form Li 2 CO 3 when discharged for long time in ambient air (reactions (3) and (4)). Although the direct reaction between O 2 − and CO 2 has been reported [32] , it is paid no attention in this study because the low CO 2 concentration (~0.03%) in ambient air and the same reaction products of Li 2 CO 3 . Owing to the distinguishable reactions, part of Li 2 O 2 and LiOH (hydration) were still in presence at the discharge termination (XRD 2). During recharging, the oxidation of the LiOH (hydration) and Li 2 O 2 happened before the Li 2 CO 3 (reactions (5)–(7)), corresponding to the two plateaus (3.6 and 4.3 V) in the charge curve ( Fig. 5 ). The higher charge overpotential related to Li 2 CO 3 decomposition is consistent with that reports on Li–O 2 batteries using carbonate-based electrolytes [12] , [33] , [34] . The recharging process sustained until the Li 2 O 2 , the LiOH (hydration) and the dominant Li 2 CO 3 almost disappeared (XRD 3), thereby ruled broadly out the degradation of the solid electrolyte and the CNG gel electrode. The Li–air cell was disassembled after charging ( Supplementary Fig. S4 ). Large amount of deposited Li metal was observed after long-period charging, while the LTAP, Celgard separator and Li metal retained stable, exhibiting efficient protection of LTAP for Li metal against dendritic contact with cathode and parasitic reactions with air. 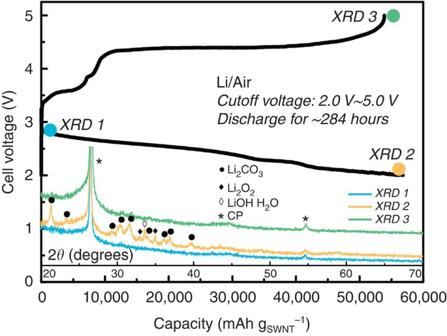Figure 5: Discharge/charge performance and XRD analysis of Li–air batteries in ambient air. Discharge/charge curves of the cell with Li salt-modified CNG. The test was carried out at 200 mA gSWNT−1in ambient air. The inset shows the corresponding XRD patterns of the CNG air electrode in its pristine state (XRD 1), after discharged to 2 V (XRD 2) and then recharged to 5 V (XRD 3). Figure 5: Discharge/charge performance and XRD analysis of Li–air batteries in ambient air. Discharge/charge curves of the cell with Li salt-modified CNG. The test was carried out at 200 mA g SWNT −1 in ambient air. The inset shows the corresponding XRD patterns of the CNG air electrode in its pristine state (XRD 1), after discharged to 2 V (XRD 2) and then recharged to 5 V (XRD 3). Full size image To evaluate the cycling performance, the Li–air cell was cycled at 200 mA g −1 in ambient air, with a fixed capacity of 2,000 mAh g −1 . Discharge/charge curves of the cell at cycles 1, 5, 25, 50 and 100 are illustrated in Fig. 6a . The discharge capacity retained 2,000 mAh g −1 over 100 cycles, while the charge capacity lowered since 30 cycles, and retained ~1,660 mAh g −1 to 100 cycles ( Fig. 6b ). The overall cycling time was over 1,880 h (~78 days). The reason of the partial and oscillating capacity decay upon charging will be discussed later through analysing the Li 2 CO 3 formation and decomposition on cycling. 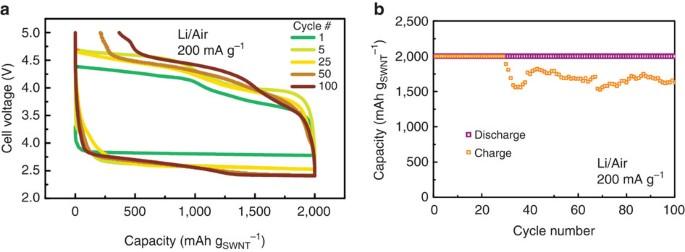Figure 6: Cycling performance of Li–air batteries in ambient air. (a) Discharge/charge curves and (b) cycling profiles of the Li–air cell with Li salt-modified CNG under a capacity limitation of 2,000 mAh gSWNT−1, and at the same time the cutoff voltages were set as 2 V for discharge and 5 V for charging. The tests were carried out in ambient air. Figure 6: Cycling performance of Li–air batteries in ambient air. ( a ) Discharge/charge curves and ( b ) cycling profiles of the Li–air cell with Li salt-modified CNG under a capacity limitation of 2,000 mAh g SWNT −1 , and at the same time the cutoff voltages were set as 2 V for discharge and 5 V for charging. The tests were carried out in ambient air. Full size image Elucidating the reversible process of Li 2 CO 3 formation and decomposition in ambient air is the key to reinforcing the understanding of the electrochemical behaviour in Li–air battery. The XRD patterns in Fig. 5 are not enough and only work for crystalline structure. Further evidence has been obtained from Fourier transform infrared (FTIR) and gas chromatography (GC) analysis. The FTIR results corresponding to Fig. 5 are illustrated in Fig. 7a . The formation and decomposition of Li 2 CO 3 is clearly identified in FTIR spectra, and no peaks associated with IL decomposition observed after both discharge and charge. For the analysis of CO 2 generated upon charging process, the GC measurement corresponding to Fig. 6 was carried out. The GC signals indicated that CO 2 gas was produced on charging ( Fig. 7b ). The measured amount of CO 2 was 0.148 ml, providing a direct evidence of Li 2 CO 3 decomposition. Herein a clear illustration corresponding to the speculated discharge/charge reactions is also given in Fig. 7c . However, we also observed that partial Li 2 CO 3 accumulated upon repetitive charging over 100 cycles ( Fig. 8 ). It is speculated that isolated Li 2 CO 3 product is in presence, which doesn’t decompose and caused the buildup of Li 2 CO 3 . The isolated Li 2 CO 3 means that separated with SWNTs during long-period cycling. We believe that the accumulation of Li 2 CO 3 is associated with the partial and oscillating capacity decay, as suggested in conventional Li–air batteries with alkyl carbonate electrolytes [3] . 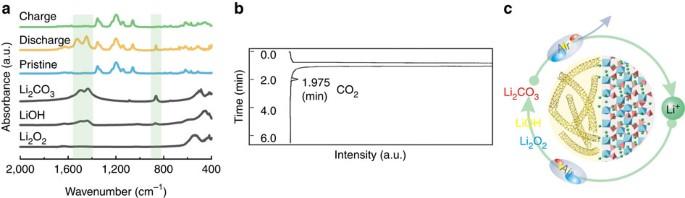Figure 7: Li2CO3formation and decomposition in ambient air. (a) FTIR spectra of a pristine cathode (Li salt-modified CNG) and after the first discharge, then charge in ambient air. The discharge/charge behaviour of the Li–air cell is corresponding toFig. 5. The reference spectra for Li2O2, LiOH and Li2CO3are also shown. (b) GC signals of CO2evolution on charging and an illustration of reversible discharge/charge process in ambient air. The GC signals were shown as a function of retention time. The analysed gas was collected at the end of the first charging process. The charging time was 10 h (2,000 mAh gSWNT−1). (c) Clear illustration of the speculated discharge/charge reactions occurring in the proposed Li–air battery in ambient air. a.u., arbitrary unit. Figure 7: Li 2 CO 3 formation and decomposition in ambient air. ( a ) FTIR spectra of a pristine cathode (Li salt-modified CNG) and after the first discharge, then charge in ambient air. The discharge/charge behaviour of the Li–air cell is corresponding to Fig. 5 . The reference spectra for Li 2 O 2 , LiOH and Li 2 CO 3 are also shown. ( b ) GC signals of CO 2 evolution on charging and an illustration of reversible discharge/charge process in ambient air. The GC signals were shown as a function of retention time. The analysed gas was collected at the end of the first charging process. The charging time was 10 h (2,000 mAh g SWNT −1 ). ( c ) Clear illustration of the speculated discharge/charge reactions occurring in the proposed Li–air battery in ambient air. a.u., arbitrary unit. 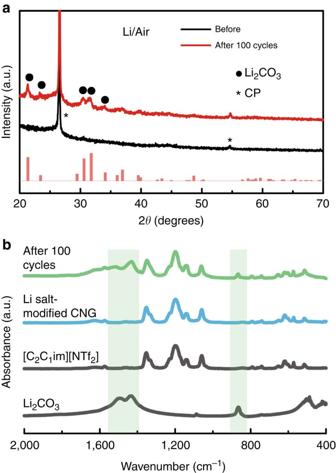Figure 8: Changes of gel cathode after 100 cycles. (a) XRD patterns of the Li salt-modified CNG cathode before and after 100 cycles in ambient air. (b) FTIR spectra of the Li salt-modified CNG electrode and the charged electrode after 100 cycles in ambient air. Both the Li salt-modified CNG cathodes used after 100 discharge/charge cycles are corresponding toFig. 6. The reference XRD pattern of Li2CO3, and the reference FTIR spectra of Li2CO3and the IL of [C2C1im][NTf2] are also shown. a.u., arbitrary unit. Full size image Figure 8: Changes of gel cathode after 100 cycles. ( a ) XRD patterns of the Li salt-modified CNG cathode before and after 100 cycles in ambient air. ( b ) FTIR spectra of the Li salt-modified CNG electrode and the charged electrode after 100 cycles in ambient air. Both the Li salt-modified CNG cathodes used after 100 discharge/charge cycles are corresponding to Fig. 6 . The reference XRD pattern of Li 2 CO 3 , and the reference FTIR spectra of Li 2 CO 3 and the IL of [C 2 C 1 im][NTf 2 ] are also shown. a.u., arbitrary unit. Full size image Conventional wisdom stated that Li–air batteries should be controlled by cutoff voltage, as well as Li-ion batteries. However, Li–air batteries represent a distinct reaction mechanism in comparison with Li-ion batteries [35] . The primary discharge product (Li 2 O 2 ) is almost completely insoluble and insulate in aprotic electrolyte. This deposition and decomposition mechanism reflects capacity fading at deep discharge because the electrode becomes blocked and deformed, as described elsewhere [36] . It is relevant here to recall two recently typical studies with cycling evaluation for Li–O 2 batteries. Sun and colleagues used the same capacity-limited test to obtain a capacity of 3,000 mAh g −1 within 50 cycles (based on the mass of carbon) [9] ; Bruce and his colleagues adopted a different cutoff voltage test to achieve a capacity of ~300 mAh g −1 for 100 cycles [11] . The latter utilized nanoporous Au as the air electrode, which was expensive but apparently more stable against electrode deformation. Therefore, the capacity-limited cycling is also an acceptable method in line with the reaction mechanism and the configuration of Li–air battery. In our case, for the first time, the Li–air cell with solid catholyte and gel air cathode has demonstrated reversible discharge–charge behaviour over 100 cycles, for a long period over 78 days and noticeably, in ambient air. In conclusion, our results demonstrate that the operation of rechargeable, long-life Li–O 2 batteries can be operated in ambient air by preventing electrolyte degradation, Li parasitic reactions with air, and dendritic short-circuit in one integrated system. The proposed Li–air cell delivered a high capacity of 56,800 mAh g −1 for discharge, as well as a high columbic efficiency of 95% for recharging during one complete cycle. The cell can further sustain repeated cycling for 100 cycles (equal to ~78 days), with a limited discharge capacity of 2,000 mAh g −1 . The discharge of Li–air battery is still based on the Li 2 O 2 formation at an electrochemical level. With air permeation, the Li 2 O 2 reacts chemically with H 2 O at first to form LiOH, and eventually reacts with CO 2 to produce Li 2 CO 3 . The recharging is a complicated process including the decomposition of Li 2 O 2 and LiOH (hydration) partially and the decomposition of Li 2 CO 3 largely, in which the latter exhibits much higher overpotential. The high overpotential will greatly affect the electrical energy efficiency of Li–air batteries. Operating Li–air batteries at higher temperature is beneficial to reduce the high overpotential ( Supplementary Fig. S5 ). At the same time, the high overpotential is reminiscent of the efforts to study the catalytic activity of transition metal oxides and precious metals on OER in carbonate-based electrolytes for Li–O 2 batteries [36] , [37] . As these catalytic activities appeared predominantly through promoting the oxidative decomposition reactions of the resultants containing Li 2 CO 3 , introducing these catalysts into the flexible gel cathode may be available for improving the electrical energy efficiency of Li–air batteries. SWNTs/IL CNG gel cathode The SWNTs/IL CNG was prepared by a method previously reported [19] , [38] . SWNTs (5 mg, Hipco SuperPure) were dispersed in 0.5 ml imidazolium ion-based IL of 1-ethyl-3-methylimidazolium bis(trifluoromethylsulfonyl)imide ([C 2 C 1 im][NTf 2 ]) by ultrasonic dispersion for 30 min. The suspension was ground in an agate mortar for 20 min. With grinding, the viscosity of SWNTs/IL suspension gradually increased, and finally forming a sticky paste. The paste was then moved to a centrifuge tube and centrifuged at 9,100 g (centrifugal force) for 3 h. The upper excess IL was removed to get the lower black SWNTs/IL crosslinked gel. The typically high-tangled SWNTs bundles were untangled upon being ground into the imidazolium ion-based [C 2 C 1 im][NTf 2 ] IL to form the gel by a possible specific interaction between the cation in [C 2 C 1 im][NTf 2 ] IL and the π-electronic nanotube surface. The as-prepared gel was pasted finely onto a carbon paper current collector. The loading area was 0.28 cm 2 . The as-prepared electrode was dried at 80 °C in vacuum for 12 h. The as-obtained air cathode has a loading weight of SWNTs as 0.8 mg cm −2 . To compare the electrochemical performance of untangled SWNTs with entangled SWNTs, the similar suspension of SWNTs and [C 2 C 1 im][NTf 2 ] by ultrasonic dispersion was centrifuged directly at 9,100 g without grinding to obtain the SWNTs/IL mixture. The Li salt-modified CNG gel was obtained by replacing the [C 2 C 1 im][NTf 2 ] IL with 0.5 M Li[NTf 2 ] salt and [C 2 C 1 im][NTf 2 ] solution during the preparation. The final Li salt-modified CNG gel contained ~0.25 M Li[NTf 2 ] salt. Solid Li conductor catholyte The lithium ion conducting solid catholyte, Li 1.35 T 1.75 Al 0.25 P 2.7 Si 0.3 O 12 (LTAP), was supplied by Ohara Inc., Japan. The preparation method of LTAP has been described elsewhere [39] , [40] . The thickness of LTAP plate was ca. 150 μm. The electrical conductivity of the LTAP plate at 25 °C was ca. 1.05 × 10 −4 S cm −1 . The XRD features of the LATP plate are mainly due to the NASICON-type LiTi 2 (PO 4 ) 3 phase, as schematically illustrated in Fig. 1 . Ethylene carbonate-based anolyte The ethylene carbonate (EC)-based anolyte consists of the Li salt of 1 M LiClO 4 , and the polar aprotic solvent of EC and diethyl carbonate (1:1 by volume). Water content in the EC-based anolyte is lower than 5 p.p.m. Li anode The Li foil with thickness of 0.2 mm was cut into a square of 8 × 8 mm, and then pressed onto Cu mesh current collector. Assembling Li–air cell All the manipulations of cell assembling were carried out in an argon-filled high-integrity glovebox. The Li anode, EC-based electrolyte and LTAP plate were sealed together compactly to make a laminated Li–air cell. A Celgard 2,400 separator was used to separate the Li metal and LTAP plate because Li metal reacts with LTAP chemically when contacting directly [41] . The EC-based anolyte was adsorbed between the Li anode and the LTAP catholyte by the Celgard separator. The SWNTs/IL CNG air cathode was pressed and fixed onto the LTAP plate directly, corresponding to the position of Li anode on the other side of the LTAP plate. The non-volatility of the gel cathode and the LTAP catholyte guarantees long-life stability of the Li–air battery in ambient air. Electrochemical measurement For the test in pure O 2 with a trace of air, the as-obtained Li–air cell was kept in a glass chamber filled with argon gas, and then took out from the glovebox. Pure O 2 flowed through the glass chamber to replace the argon gas, in the meantime, the O 2 valve was adjusted to allow a trace of air permeance. The indication of air permeance was the colour change of a piece of Li foil put in the glass chamber in advance from silver to black and then a little white gradually. For the test in air, the as-obtained Li–air cell was put in the ambient air directly. All the tests were carried out under a gas pressure of 1 atm. All of the current densities were constant at 200 mA g SWNT −1 (0.16 mA cm −2 ). The electrochemical tests were performed at 25 °C using Hokuto charge/discharge machine and Solartron instruments. The capacity was normalized by the weight of the SWNTs. The anchored IL is considerably stable during long-period operation in air, as shown in Fig. 8 . The current collector of carbon paper has been confirmed no contribution to discharge ( Supplementary Fig. S6 ). How to cite this article: Zhang, T. and Zhou, H. A reversible long-life lithium-air battery in ambient air. Nat. Commun . 4:1817 doi: 10.1038/ncomms2855 (2013).